Relativistic frequency upshift to the extreme ultraviolet regime using self-induced oscillatory flying mirrors Coherent short-wavelength radiation from laser–plasma interactions is of increasing interest in disciplines including ultrafast biomolecular imaging and attosecond physics. Using solid targets instead of atomic gases could enable the generation of coherent extreme ultraviolet radiation with higher energy and more energetic photons. Here we present the generation of extreme ultraviolet radiation through coherent high-harmonic generation from self-induced oscillatory flying mirrors—a new-generation mechanism established in a long underdense plasma on a solid target. Using a 30-fs, 100-TW Ti:sapphire laser, we obtain wavelengths as short as 4.9 nm for an optimized level of amplified spontaneous emission. Particle-in-cell simulations show that oscillatory flying electron nanosheets form in a long underdense plasma, and suggest that the high-harmonic generation is caused by reflection of the laser pulse from electron nanosheets. We expect this extreme ultraviolet radiation to be valuable in realizing a compact X-ray instrument for research in biomolecular imaging and attosecond physics. Coherent short-wavelength radiation is crucial for research pertaining to ultrafast electron dynamics in atoms, molecules, plasmas and solids. To date, various physical mechanisms based on laser–plasma interactions, such as plasma-based X-ray lasers [1] , [2] , nonlinear Thomson scattering [3] , betatron radiation [4] , relativistic flying mirrors [5] , X-ray-free electron lasers [6] and high-order harmonics (HOH) [7] , [8] have been investigated in attempts to produce ultrafast short-wavelength radiation in the extreme ultraviolet (XUV) range. Among these approaches, high-harmonic generation (HHG) from gaseous targets has been extensively studied to produce a bright attosecond XUV radiation source in the multi-keV region. To date, generation of the shortest wavelength, corresponding to ∼ 1.6 keV (ref. 9 ), was reported by focusing mid-infrared femtosecond laser pulses on gaseous targets. HHG from gaseous targets has been described by the electron recollision process [10] , and the cut-off frequency of the HOH is restricted by the ionization effect. Thus, the intensity typically used ranges from 10 14 to 10 16 W cm −2 . An alternative approach for producing a bright attosecond XUV source is to use relativistic or nonrelativistic laser-plasma on solid targets at a higher intensity. In this case, the cut-off frequency is not restricted by the ionization effect, but determined by physical conditions such as the irradiated intensity and the plasma density. Two different mechanisms, coherent wake emission (CWE) [11] and the relativistic oscillating mirror (ROM) [12] , [13] , have been proposed to explain HHG from solid targets. In the CWE mechanism, phase matching between the electromagnetic field and plasma oscillations in a density gradient leads to the emission of harmonics up to the plasma frequency. In the ROM mechanism, on the other hand, the HOH result from the reflection of the incident laser pulse due to the relativistically oscillating plasma surface. In this case, a very high temporal contrast should be applied to produce a steep plasma density gradient on the solid target [12] , [13] . Here the oscillating plasma surface with a short density-scale length ( L / λ «1) acts as a ROM [14] , [15] , and the harmonics generated from the ROM are phase-locked [16] , forming attosecond pulses. Note that the highest harmonic order in the ROM mechanism is proportional to γ 3 (where γ is the Lorentz factor), whereas the order in the CWE is limited by the maximum plasma frequency of the target. In 2006, HHG utilizing this ROM mechanism was successfully demonstrated in the water window region (2.3–4.4 nm) through the use of a sub-picosecond petawatt Nd:glass laser system [12] , and later extended to the multi-keV regime by further increasing the laser energy on the target [13] . In this article, we report on a new mechanism for generating XUV radiation through HHG from solid targets. In contrast to a ROM mechanism that requires high-contrast (10 −10 –10 −11 ) laser pulses to realize a short density-scale length [12] , [13] , [17] , [18] , the new mechanism reveals that in a long underdense plasma ( L / λ »1), the formation of relativistically oscillating and flying electron nanosheets is possible and that an incident laser frequency can be upshifted to the XUV range using electron nanosheets. To experimentally realize this mechanism, an appropriate plasma density-scale length should be exploited by adjusting the temporal contrast between the main pulse and an amplified spontaneous emission (ASE). We then carry out particle-in-cell (PIC) simulations to theoretically explain our mechanism and experimental results. In brief, a plasma having a long scale length of ∼ 100 μm, measured using an interferometer, can be induced by a certain level of ASE intensity on a solid target, which supports the multiple formation of oscillatory flying electron nanosheets in a propagating laser pulse: these electron nanosheets act as oscillatory flying mirrors (OFMs; see Fig. 1 ). Although the oscillating motion of electron nanosheets provides a high degree of periodicity to the laser field cycle and results in HHG, the HOH generated by the OFM mechanism are not strictly periodic to the laser field cycle because of the forward and backward motions of the electron nanosheets. In this sense, the HOH generated by the OFM mechanism is distinct from conventional relativistic harmonics obtained by ROM. Here we could obtain a short wavelength of up to 4.9 nm by focusing a 30-fs, 10-Hz, 100-TW Ti:sapphire laser pulse on a solid target. As such, these experimental results are the first demonstration of a relativistic frequency upshift for generating XUV radiation through an OFM mechanism working in a long underdense plasma. 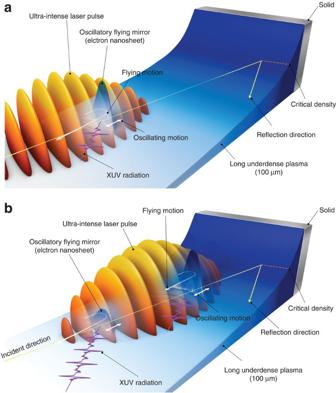Figure 1: Formation of OFMs and XUV radiation in a long underdense plasma. (a) In a long underdense plasma, a high-density electron nanosheet is built up in the leading edge of a propagating ultraintense laser pulse. This electron nanosheet acts as an OFM reflecting the incident laser pulse and, consequently, XUV radiation is generated in the direction of the reflection. (b) Multiple OFMs are built up during the propagation of the laser pulse through the underdense plasma. The ultrafast flying motion of an electron nanosheet significantly extends the generated XUV spectrum to a shorter wavelength. Figure 1: Formation of OFMs and XUV radiation in a long underdense plasma. ( a ) In a long underdense plasma, a high-density electron nanosheet is built up in the leading edge of a propagating ultraintense laser pulse. This electron nanosheet acts as an OFM reflecting the incident laser pulse and, consequently, XUV radiation is generated in the direction of the reflection. ( b ) Multiple OFMs are built up during the propagation of the laser pulse through the underdense plasma. The ultrafast flying motion of an electron nanosheet significantly extends the generated XUV spectrum to a shorter wavelength. Full size image Experimental results We first performed the generation of HOH from solid targets using high-contrast laser pulses. Previous studies [12] , [13] , [17] , [18] have shown that these laser pulses were essential for generating XUV radiation through relativistic HHG from solid targets. In this case, the power scaling law for the harmonic spectrum is given by n −8/3 (where n is the harmonic order), and the cut-off for the maximum harmonic order is given by 8 1/2 γ 3 ( [19] ). 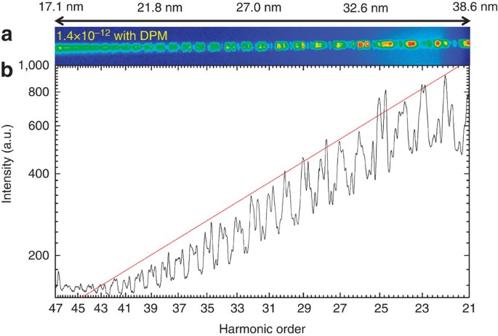Figure 2: HOH spectrum obtained with DPM. (a) Raw charge-coupled device (CCD) image of the spectral range between 17.1 and 38.6 nm obtained using two 0.2-μm thick Al filters. (b) Harmonic spectrum ofaon a logarithmic scale. These harmonic spectra are shown after correcting for the factors that affect the spectral sensitivity, such as the transmission of Al filters, reflectivity of the toroidal mirror, diffraction efficiency of the concave grating and quantum efficiency of the X-ray CCD in the flat-field XUV spectrometer. The red line represents the power scaling ofn−8/3for the harmonic spectrum. Figure 2 shows the HOH spectrum measured using a SiO 2 solid target and a high-contrast laser pulse. The peak intensity on the target obtained with a double plasma mirror (DPM) system was 4.5 × 10 19 W cm −2 . The DPM system was used to reach a temporal contrast of 1.4 × 10 –12 at 500 ps before the main pulse. In our experiments using high-contrast laser pulses, the power scaling for the harmonic spectrum agreed well with an n −8/3 dependence, and the cut-off was determined to be at the 43rd order (18.7 nm). This result, obtained with a high-contrast laser pulse, is similar to those previously reported by other groups [20] . Figure 2: HOH spectrum obtained with DPM. ( a ) Raw charge-coupled device (CCD) image of the spectral range between 17.1 and 38.6 nm obtained using two 0.2-μm thick Al filters. ( b ) Harmonic spectrum of a on a logarithmic scale. These harmonic spectra are shown after correcting for the factors that affect the spectral sensitivity, such as the transmission of Al filters, reflectivity of the toroidal mirror, diffraction efficiency of the concave grating and quantum efficiency of the X-ray CCD in the flat-field XUV spectrometer. The red line represents the power scaling of n −8/3 for the harmonic spectrum. Full size image On the other hand, shorter-wavelength XUV radiation could be obtained with higher harmonic orders when the contrast ratio of the laser pulses was carefully optimized. 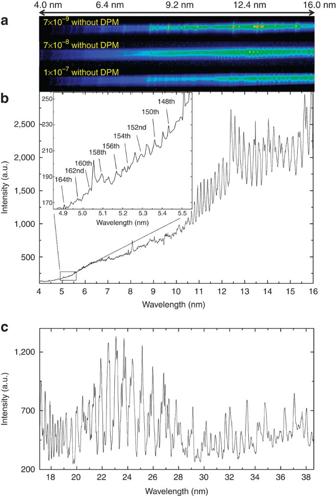Figure 3: HOH spectra obtained with different temporal contrasts. The DPM was removed and the ASE level was controlled by adjusting the switching-on time of a UPC. (a) Raw CCD images in the spectral range between 4 and 16 nm obtained using two 0.1-μm thick Ti filters. (b) Harmonic spectrum ofaat a contrast of 7 × 10–8at 500 ps before the arrival of the main laser pulse. (c) Harmonic spectrum in the spectral range between 17.1 and 38.6 nm obtained using two 0.2-μm thick Al filters at a contrast of 7 × 10–8. Here it is clearly shown that the harmonic spectrum does not follow the power scaling law (n−8/3). Figure 3 shows the HOH spectra when the temporal contrast of the laser pulses was controlled using an ultrafast Pockels cell (UPC); no DPM system was used in this case. Here the contrast ratio varied from 7 × 10 –9 to 1 × 10 –7 by adjusting the switch-on time of the UPC at 500 ps before the main pulse. In our experiments, the highest-order harmonic signal was obtained at 4.9 nm (the 164th order) when the optimum contrast ratio of 7.0 × 10 –8 was found, as shown in Fig. 3b . Note that the harmonic signal above the 100th order became weaker as the contrast ratio differed from the optimum value. In addition, the figure shows that harmonics shorter than 4.9 nm could not be clearly distinguished from the atomic emission lines of Si and O atoms (see also Supplementary Fig. S1 ), and that a weak and continuous spectrum was observed because of the low detection efficiency and low resolving power of the XUV spectrometer optimized at 10 nm. At a peak laser intensity of 4.5 × 10 19 W cm −2 , comparable to that of a DPM system, HOH up to the 129th order (6.2 nm) was clearly observable. Moreover, the harmonic spectra obtained without the DPM system showed different characteristics (in terms of power scaling law and cut-off frequency) from the well-known relation given by the ROM model. For example, the high-harmonic signal did not follow the power scaling law n −8/3 at all; rather, the harmonic spectrum longer than 12 nm was modulated, as shown in Fig. 3b . The differences in the spectral characteristics of the harmonics between the high-contrast and optimized-contrast cases may be explained by the presence of plasma with a long density-scale length. Figure 3: HOH spectra obtained with different temporal contrasts. The DPM was removed and the ASE level was controlled by adjusting the switching-on time of a UPC. ( a ) Raw CCD images in the spectral range between 4 and 16 nm obtained using two 0.1-μm thick Ti filters. ( b ) Harmonic spectrum of a at a contrast of 7 × 10 –8 at 500 ps before the arrival of the main laser pulse. ( c ) Harmonic spectrum in the spectral range between 17.1 and 38.6 nm obtained using two 0.2-μm thick Al filters at a contrast of 7 × 10 –8 . Here it is clearly shown that the harmonic spectrum does not follow the power scaling law ( n −8/3 ). Full size image To verify the presence of this plasma, we measured the electron-density profile using an interferometer. 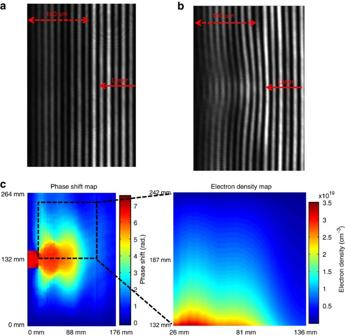Figure 4: Measurement of electron-density profile using an interferometer. Interferograms recorded using a 400-nm probe beam were taken at 50 ps before the main laser pulse (a) with DPM (1.4 × 10−12) and (b) without DPM (7 × 10−8). (c) Electron-density profile ofb. Figure 4 presents the interferogram measured with underdense plasma under high-contrast (1.4 × 10 –12 , with DPM) and optimized-contrast (7 × 10 –8 , without DPM) laser pulse conditions. The interferogram was taken using a 400-nm probe beam at 50 ps before the main laser pulse. The pixel resolution of the CCD (1,280 × 1,024) was 0.44 μm. For the high-contrast laser pulse, no noticeable underdense plasma was observed (see Fig. 4a ), showing straight interference lines. On the other hand, for the optimized-contrast laser pulse, the formation of an underdense plasma with a long density-scale length was clearly observed (see Fig. 4b ). Figure 4c then shows the electron-density profile of the underdense plasma calculated from the interferogram obtained using an optimized-contrast laser pulse. From Fig. 4c , the calculated plasma density-scale length was about 100 μm. Figure 4: Measurement of electron-density profile using an interferometer. Interferograms recorded using a 400-nm probe beam were taken at 50 ps before the main laser pulse ( a ) with DPM (1.4 × 10 −12 ) and ( b ) without DPM (7 × 10 −8 ). ( c ) Electron-density profile of b . Full size image Several interesting features were observed in the harmonic spectra measured in our experiments. For example, spectral splitting (or broadening) was observed in many harmonic orders for both high-contrast and optimized-contrast laser pulses, though spectral splitting in the harmonic order generated by high-contrast laser pulses has already been reported by other groups [20] , [21] . According to previous studies, spectral splitting is related to the ultrafast oscillatory surface motion of electrons. In our experiments using optimized-contrast laser pulses, both a spectral shift, defined by Δ ω n / ω n (where Δ ω n is the frequency shift of the n -th harmonic with frequency ω n ), as well as spectral splitting were observed in the harmonic spectrum. 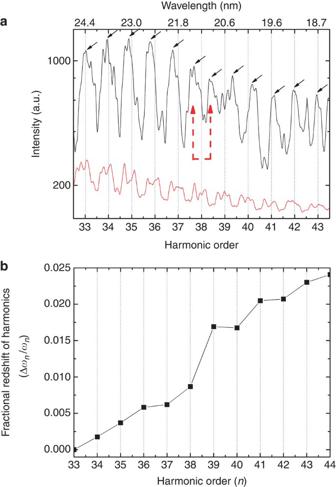Figure 5: Spectral redshift of HOH obtained without DPM. (a) HOH spectrum obtained with (red line) and without (black line) DPM on a logarithmic scale. The average spectral spacing between harmonic orders obtained without DPM can be expressed as 0.96 × (ωn+1−ωn), whereωnis the frequency of then-th harmonic order. An abrupt jump of 0.67 × (ωn+1−ωn) in the redshift between the 38th and 39th orders is observed as shown by red dashed two arrows. (b) Fractional redshift of harmonic lines (Δωn/ωn, where Δωnis the frequency shift of then-th harmonic with frequencyωn) obtained at a contrast of 7 × 10−8without DPM. Figure 5a shows the harmonic spectra in the range of 18.5–24.8 nm obtained using high-contrast and optimized-contrast laser pulses. In the figure, a spectral redshift for the optimized-contrast laser pulses can be seen, whereas the central position of each harmonic line for the high-contrast laser pulse was located at the position of an integer harmonic order. In this spectral range, 12 harmonic lines are counted for the optimized-contrast laser pulse, whereas 11 harmonic lines are seen for the high-contrast laser pulse. Figure 5: Spectral redshift of HOH obtained without DPM. ( a ) HOH spectrum obtained with (red line) and without (black line) DPM on a logarithmic scale. The average spectral spacing between harmonic orders obtained without DPM can be expressed as 0.96 × ( ω n +1 − ω n ), where ω n is the frequency of the n -th harmonic order. An abrupt jump of 0.67 × ( ω n +1 − ω n ) in the redshift between the 38th and 39th orders is observed as shown by red dashed two arrows. ( b ) Fractional redshift of harmonic lines (Δ ω n / ω n , where Δ ω n is the frequency shift of the n -th harmonic with frequency ω n ) obtained at a contrast of 7 × 10 −8 without DPM. Full size image Figure 5b shows the amount of spectral redshift as a function of harmonic order. The average spectral spacing between harmonic orders was 0.96 × ( ω n +1 − ω n ), where ω n is the frequency of the n -th harmonic order). Interestingly, we also observed an abrupt jump of 0.67 × ( ω n +1 − ω n ) in the redshift between the 38th and 39th orders because of the transition from integer harmonics to half-integer harmonics (see also Supplementary Fig. S2 ), which is similar to that shown in Fig. 4d of (ref. 20 ). Although only the redshift is shown in Fig. 5 , both a blueshift and a redshift were observed at higher harmonic orders (see Supplementary Figs S3 and S4 ), possibly related to the co- and counter-propagating motion of electron nanosheets in a long underdense plasma, although further investigations pertaining to the redshift and blueshift should be performed through theoretical and experimental studies. Consequently, these spectral characteristics distinguished the harmonic spectrum obtained using an optimized-contrast laser pulse from the relativistic HOH obtained by a conventional ROM. Relativistic HHG using ROM model We performed one-dimensional and two-dimensional PIC simulations using the APRI laser plasma simulator (ALPS) code [22] , [23] to theoretically explain the experimental results. 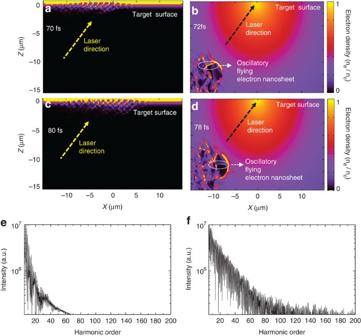Figure 6: The two-dimensional PIC simulation results for generating HOH. Evolution of electron densities in sharp plasma density (a,c) and long plasma density (b,d) regimes. High-harmonic spectra from a solid target obtained for (e) the high-contrast case and for (f) the optimized-contrast case are shown. Figure 6 shows the results for a simulation of the solid targets with both a sharp plasma density and a long plasma density. For the target with the sharp plasma density, the reflection surface oscillated as explained by the ROM model. In brief, relativistic electrons are periodically pulled from the target surface by the laser pulse (see Fig. 6a ) and the laser pulse is reflected by these high-speed dense electrons, resulting in XUV radiation through the HHG process. The harmonic spectrum obtained in this case is shown in Fig. 6e , and follows the power scaling law of n −8/3 ; the cut-off of the harmonic order was about the 50th order. This simulation result agreed well with the experimental and numerical results reported by other groups [13] , [19] . Figure 6: The two-dimensional PIC simulation results for generating HOH. Evolution of electron densities in sharp plasma density ( a , c ) and long plasma density ( b , d ) regimes. High-harmonic spectra from a solid target obtained for ( e ) the high-contrast case and for ( f ) the optimized-contrast case are shown. Full size image Formation of OFM using optimized-contrast laser pulses For the target with the long underdense plasma density, however, the harmonic spectrum generation process was different from that explained in the ROM model. During the laser propagation through the long underdense plasma, background electrons were pushed forward by the ponderomotive force of the laser pulse and formed a co-propagating high-density spike (electron nanosheet) in the leading edge of the laser pulse (see Fig. 6b ). The laser pulse was partly reflected by the co-propagating oscillatory electron nanosheet, resulting in a spectral redshift at low harmonic orders. Then, at some point, the co-propagating electron nanosheet was stopped by the space charge force and began a backward (counter-propagating) oscillatory motion due to the ponderomotive force with the reverse sign. Within a short time period, the electron nanosheet attained a speed close to the speed of light in vacuum (see Fig. 6b ). Consequently, the incident laser pulse was reflected by the relativistically oscillating and flying electron nanosheet, which formed an OFM. After a few oscillation periods, the counter-propagating electron nanosheet smeared out into the background plasma, while at the same time a portion of the incident laser pulse propagated into the higher-density region and initiated the creation of another electron nanosheet at a different position (see Supplementary Fig. S5 ). XUV radiation through HHG by OFM model The harmonic spectrum generated by the OFM mechanism is shown in Fig. 6f . The spectrum calculated using the optimized-contrast case extended to over the 200th order and showed a stronger signal than that of the high-contrast case at higher harmonics above the 10th order. We then calculated the speed and the Lorentz factor γ of an electron nanosheet to explain the extension of the harmonic order to the shorter wavelength. In PIC simulations, the average speed ( v >0.6 c ) of the electron nanosheet formed in the long underdense plasma was much higher than used in (ref. 19 ), which was obtained using a sharp plasma density. Here the γ factor became as high as 25 in a short time (about half of the laser period); consequently, the extension of harmonic orders to the shorter wavelength is related to the high speed of the electron nanosheet. In principle, attosecond pulse generation is possible by filtering an appropriate bandwidth from the obtained harmonic spectrum (see Supplementary Fig. S6 ). However, further investigation is required to accurately characterize temporal properties such as the pulse duration and profile. By using a self-induced OFM mechanism, we have demonstrated the generation of XUV radiation through a coherent HHG process in a long underdense plasma. The simulation results obtained here indicate that the ultrafast oscillatory and flying motion of an electron nanosheet formed in a long underdense plasma was responsible for producing the XUV radiation. To realize the OFM mechanism, the plasma density-scale length was optimized by adjusting the temporal contrast between the main pulse and an ASE. We then successfully generated XUV radiation up to 4.9 nm through the self-induced OFM. In practical applications, short-wavelength generation through the OFM mechanism will be a great advantage, because the OFM mechanism does not require any contrast enhancement device, such as a plasma mirror system. In addition, by using a recently developed petawatt Ti:sapphire laser [24] , [25] with an optimized temporal contrast, repetitive and efficient generation of bright and coherent XUV in the water window or the multi-keV region should be possible. Indeed, it is expected that the extension to shorter wavelength will enable the production of bright attosecond pulses in the water window range and beyond, thereby boosting the ability of attosecond science to investigate ultrafast atomic and molecular dynamics and life science to explore biomolecular dynamics using ultrafast X-ray imaging techniques. Experimental methods The CPA Ti:sapphire laser system (10 Hz, 30 fs, 100 TW) at the Advanced Photonics Research Institute was used to efficiently generate HOH signals from solid targets. Supplementary Figure S7 shows the experimental setup for generating HOH signals from a solid target. In brief, a 30-fs (fundamental wavelength 805 nm) laser pulse with 2 J in energy and a 70-mm beam diameter was delivered to a DPM system to ensure a high-contrast laser pulse (see Supplementary Fig. S7a ). In the DPM system, the laser pulse was focused with an off-axis parabolic (OAP) mirror, and its focal plane was located at the midpoint between two antireflection-coated plasma mirrors. After reflection from a second plasma mirror, the laser beam was collimated by another OAP mirror; the beam size was then increased to its original diameter before the beam was directed into the target chamber. A translation stage before the DPM made it possible to directly deliver laser pulses to the target chamber without the DPM system, when necessary. The features of the DPM system are described in detail elsewhere [26] . After the DPM system, the p-polarized laser beam was focused on the target using an OAP mirror ( f =25 cm) at an incident angle of 45° (see Supplementary Fig. S7b ). The final laser pulse energy on the target was 2 J without the DPM system and 1 J with the DPM system. HOH spectra were then observed using a flat-field XUV spectrometer installed along the optical axis of the beam reflected from the solid target. The spectrometer consisted of a gold-coated toroidal mirror, a 1,200 lines per mm grating (Hitachi), X-ray filters and a back-illuminated X-ray CCD (Princeton Instruments, PI-SX:2K). The spectrometer was calibrated with an aluminium (Al) L-edge (17.1 nm), and its second order (34.2 nm) observed from the atomic emission lines (see Supplementary Fig. S8 ). Polished SiO 2 was chosen as the solid target for HOH generation, and the surface roughness of the target was a few nanometer (less than 10 nm) in root-mean-square value. Supplementary Figure S9a,b shows the focal spot images of the laser beam measured with and without the DPM system, respectively. At an energy fluence of 90 J cm −2 in the DPM system, the focusability of the laser beam was not seriously affected; thus, the focal spot size and its shape measured with the DPM system were similar to those measured without the DPM system. The measured focal spot size was a 5 μm at full-width at half-maximum in both the vertical and horizontal directions, and the calculated energy concentration within the full-width at half-maximum was around 50%. Consequently, the peak intensity on the target was 9 × 10 19 W cm −2 without the DPM system, and 4.5 × 10 19 W cm −2 with the DPM system. The temporal contrast of the laser pulse was then measured using a third-order cross-correlator (Amplitude Technologies, SEQUOIA); the contrast ratio measurement, up to 500 ps before the main pulse, is shown in Supplementary Fig. S10 . The measured contrast ratios at 500 ps before the main pulse were 1.4 × 10 –12 (high-contrast case) and 7 × 10 –8 (optimized-contrast case) with and without the DPM system, respectively. Thus, the contrast enhancement with the DPM system was better than 10 4 . In the experiment without the DPM system, the temporal contrast was adjusted by controlling the switch-on time of a UPC that was installed in front of the pulse stretcher and was used to increase or decrease the ASE level of the laser pulses. PIC simulation Using 1D- and 2D-PIC simulations, we investigated the generation of high harmonics under two target conditions: a solid target with a sharp plasma density (a density-scale length of L / λ «1 was assumed for the high-contrast laser case) and a solid target with a long plasma density (80-μm-long underdense plasma for the optimized-contrast (7 × 10 –8 ) laser case). The plasma density-scale length of 80 μm was chosen by considering the experimentally measured plasma density-scale length and taking into account the memory capacity and computing time. For the two-dimensional PIC simulations, a spherically symmetric electron-density profile in front of the target surface was assumed before the arrival of the main pulse. In all simulations, a p-polarized laser pulse with a normalized amplitude a 0 of 6.5 (4.6 for the high-contrast case) and a pulse duration of 30 fs was launched into the solid target at an angle of 45°. The validity of the ALPS code used in our simulations has been demonstrated in other studies [22] , [23] . How to cite this article: Kim, I. J. et al. Relativistic frequency upshift to the extreme ultraviolet regime using self-induced oscillatory flying mirrors. Nat. Commun. 3:1231 doi: 10.1038/ncomms2245 (2012).